Dispersant-free conducting pastes for flexible and printed nanocarbon electrodes The dispersant-free fabrication of highly conducting pastes based on organic solvents with nanocarbon materials such as carbon nanotubes and graphene nanoplatelets has been hindered by severe agglomeration. Here we report a straightforward method for fabricating nanocarbon suspensions with >10% weight concentrations in absence of organic dispersants. The method involves introducing supramolecular quadruple hydrogen-bonding motifs into the nanocarbon materials without sacrificing the electrical conductivity. Printed films of these materials show high electrical conductivity of ~500,000 S m −1 by hybridization with 5 vol% silver nanowires. In addition, the printed nanocarbon electrodes provide high-performance alternatives to the platinum catalytic electrodes commonly used in dye-sensitized solar cells and electrochemical electrodes in supercapacitors. The judicious use of supramolecular interactions allows fabrication of printable, spinnable and chemically compatible conducting pastes with high-quality nanocarbon materials, useful in flexible electronics and textile electronics. Highly concentrated colloidal suspensions of nanocarbon (NC) materials are of great interest for a variety of applications, ranging from flexible electronics and flexible conducting fibres to electrochemical electrodes for energy-harvesting or storage devices [1] , [2] , [3] , [4] , [5] , [6] , [7] . Direct printing technologies using printable NC-conducting pastes with high conductivity and flexibility can be expected to show promise in the development of emerging flexible electronics. However, one of the key technical challenges in NC material science is to overcome the difficulties associated with processing such NC materials for further applications. Unfortunately, unless the NC materials are highly functionalized with oxidative moieties or are shortened using ball milling, they agglomerate irreversibly at weight concentrations >1.0 wt% because of their high aspect ratio (>500) and strong van der Waals attraction, making further processing difficult [8] . However, such severe covalent functionalization of NC materials inevitably degrades their electrical and/or electronic properties to some degree [9] , [10] . Thus, many additives such as organic surfactants [11] , alkali solutions [12] , superacids [1] , [2] , N -methylpyrrolidone (NMP) [13] and ionic liquids [4] have been used to prepare highly concentrated NC suspensions. A disadvantage of this approach is that the overall properties (for example, the electrical and thermal properties) of the mixtures can suffer because of high intertube or sheet-to-sheet junction resistance because the conducting nanomaterials may be separated by the insulating organic materials added to facilitate dispersion and processing. In the case of superacids, although they have been successfully used to dissolve carbon nanotubes (CNTs) and exfoliate graphite for bulk processing, they have the drawback of chemical incompatibility with other materials, which prevents diverse applications. Here we show that quadruple hydrogen bond networks can overcome these issues for fabricating printable, spinnable and chemically compatible conducting pastes containing high-quality CNTs and graphene nanoplatelets in organic solvents without the need for additional dispersion agents. The shear-thickening behaviour of our NC pastes and the unusual drying behaviour of the diluted NC suspension droplet provide rheological and colloidal evidence of the presence of multiple strong noncovalent bonds. The dispersant-free pastes could form rationally designed hybridized materials including polymers, metals and metal oxides. In particular, the printed supramolecular CNTs/Ag nanowire (NW) hybrid film has a high electrical conductivity of~500,000 S m −1 . The practical value of such strategies is demonstrated by successfully using printed multiwalled CNT (MWNT) and single-walled CNT (SWNT)/graphene hybrid coatings as high-performance electrochemical electrodes in a dye-sensitized solar cell (DSC) and in an electrochemical capacitor, respectively. Synthesis of NC materials with quadruple hydrogen-bonding motifs The specific set of hydrogen bonds formed has an important role in determining the three-dimensional structure of chemical and biological systems because of the bonds’ specificity and directionality [14] , [15] , [16] . Motivated by the self-assembly of donor–donor–acceptor–acceptor arrays of hydrogen-bonding sites [15] , we functionalized NC materials with 2-ureido-4[1H]pyrimidinone (UHP) moieties forming quadruple hydrogen bonding (QHB) to overcome their severe van der Waals attraction ( Fig. 1a ). QHB arrays are much stronger than triple hydrogen-bond arrays and are easily accessible synthetically. The dimerization constants of donor–donor–acceptor–acceptor arrays of UHP moieties (>10 7 M −1 in chloroform) are 2–3 orders of magnitude higher than that (>10 5 M −1 ) found for the synthetically less accessible AAA and DDD arrays [17] . The supramolecular NCs (supra-NCs) modified with UHP moieties were synthesized in three steps from commercially available starting materials. NC materials functionalized with carboxylic acid groups were sequentially reacted with toluene diisocyanate (TDI) and 2-amino-4-hydroxy-6-methyl-pyrimidine (AHMP) to attach the isocyanate and UHP groups, respectively ( Fig. 1a ). The chemical structure of pristine NCs, carboxylated NCs (NC-COOH), isocyanate-functionalized NCs and supra-NCs with QHB motifs were characterized by X-ray photoelectron spectroscopy (XPS) and Fourier transform infrared (FTIR) spectroscopy ( Supplementary Figs S1–S4 ). The band at 1,705 cm –1 in the FTIR spectra indicated the presence of carboxylic acid groups. This band disappeared and an isocyanate peak (2,270 cm –1 ) appeared after the coupling reaction with TDI. Importantly, amide bonds (1,680 cm –1 ) and broad hydrogen peaks were observed after the coupling reaction with AHMP. An N1s peak, which was absent from the XPS spectra of MWNT-COOH, appeared in the XPS spectra of the supra-MWNTs ( Supplementary Fig. S4 ). 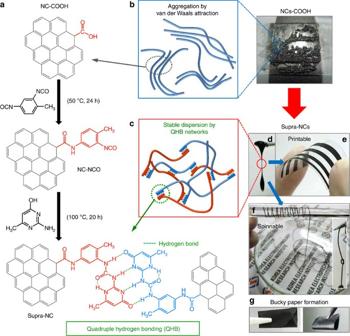Figure 1: Dispersant-free formation of NC-based conducting pastes. (a) Synthetic scheme for supra-NCs, in which CNTs functionalized with carboxylic acid groups using a HNO3/H2SO4mixture (1/3, v/v), such as MWNTs-COOH, SWNTs-COOH and graphene oxide nanoplatelets, were sequentially reacted with TDI and AHMP to form UHP moieties. (b) Schematic illustration and photograph of an unstable colloidal suspension of NCs-COOH prepared without a dispersant. (c) Schematic illustration of a stable supra-NC paste. (d) Photographs of the supra-NC paste drop. (e) The printed film on the plastic substrate. (f) The conductive fibre with a high supra-SWNT content (~70 wt%). (g) Bucky papers with supra-SWNTs (left) and long supra-MWNTs/Ag NWs (right). Figure 1: Dispersant-free formation of NC-based conducting pastes. ( a ) Synthetic scheme for supra-NCs, in which CNTs functionalized with carboxylic acid groups using a HNO 3 /H 2 SO 4 mixture (1/3, v/v), such as MWNTs-COOH, SWNTs-COOH and graphene oxide nanoplatelets, were sequentially reacted with TDI and AHMP to form UHP moieties. ( b ) Schematic illustration and photograph of an unstable colloidal suspension of NCs-COOH prepared without a dispersant. ( c ) Schematic illustration of a stable supra-NC paste. ( d ) Photographs of the supra-NC paste drop. ( e ) The printed film on the plastic substrate. ( f ) The conductive fibre with a high supra-SWNT content (~70 wt%). ( g ) Bucky papers with supra-SWNTs (left) and long supra-MWNTs/Ag NWs (right). Full size image Fabrication and characterization of dispersant-free NC pastes Figure 1b,c illustrates the striking synergy developed by introducing UHP-based QHB motifs into NC materials for the fabrication of dispersant-free supra-NC pastes. We could not prepare an NC paste using NCs functionalized solely with carboxylic acid in organic solvents because severe agglomeration occurred because of the strong van der Waals attraction in the absence of a dispersant ( Fig. 1b ). However, our approach involving the formation of a supramolecular QHB network based on UHP groups yielded well-dispersed pastes with fluid surface tensions that were so sufficiently low that the pastes could be spread over a wide range of substrates yet high enough to prevent colloidal agglomeration after deposition ( Fig. 1c ). It is worth noting that over 10 wt% colloidal suspensions of the supra-NCs interconnected with QHB motifs formed well-dispersed pastes even with long MWNTs (length >100 μm) when they were simply stirred in common solvents such as dimethylformamide (DMF) and NMP ( Fig. 1d ). These unique pastes were printable, spinnable and could be formed into flexible bucky paper by performing casting or filtration. To confirm that NC materials form QHB networks in the colloidal suspension, we investigated the shear rate dependence of the viscosity for the supra-NC pastes. Usually, in hard-sphere colloidal suspensions, the low-shear viscosity increases when the volume fraction is increased beyond ~50%, and shear thickening or a jamming transition may occur [18] , [19] . This behaviour depends on the nature of the particle–particle interactions [19] . Notably, in this study, we observed shear thickening in the low-shear regime even at concentrations below 10% ( Fig. 2a ). These results clearly indicate that the supra-NC materials are interconnected by strong interactions among the CNTs and graphene nanoplatelets functionalized with QHB motifs. Moreover, from diluted supra-NC suspensions, we also observed the unusual drying patterns of the supra-NC droplets on the substrate due to QHB networks, which are in stark contrast to the acid-treated NCs ( Fig. 2b,c ). The droplet of MWNT-COOH nanocolloids dried at 20 °C tended to leave a typical coffee-ring drying pattern typical of water-soluble or dispersible materials ( Fig. 2b ) [20] . The suspended particles tend to move towards the edges of the droplet during solvent evaporation because the solvent evaporation rate of DMF is low at 20 °C and is highest at the edge of the droplet, which induces fluid flow towards the edge. By contrast, supra-MWNTs became agglomerated in the centre of the droplet during drying at 20 °C, indicating that MWNTs interconnected by QHB motifs behave as macro particles and cannot move towards the edges of the droplet, which can be explained by the diffusion-limited aggregation model [21] . Supra-SWNTs and supra-reduced graphene oxide (RGO) showed similar fluid properties. Interestingly, the reverse evaporation behaviour was observed at 100 °C, at which the amplified temperature gradient induces Marangoni flow [22] . MWNTs-COOH left residues in the centre of the droplet because of the Marangoni flow, whereas clear coffee rings were observed in the supra-MWNT droplets ( Fig. 2c ). The interconnected supra-MWNTs supported a weak Marangoni flow even at high temperatures. Therefore, our observations suggest that most of the supra-NCs were interconnected by multiple strong hydrogen bonds in the suspension. 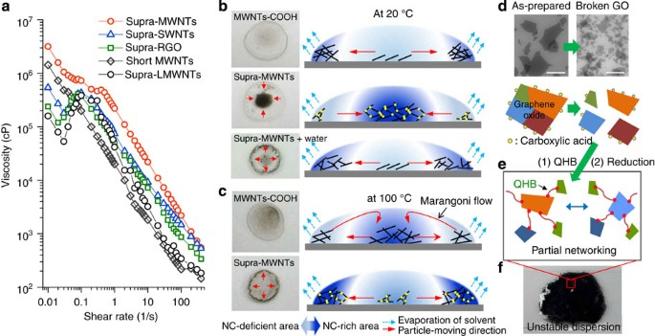Figure 2: Rheological and colloidal evidence of network formation. (a) Shear viscosity plot for supra-NC pastes (~10 wt%) in DMF as a function of shear rate showing shear-thickening behaviour at a low shear rate. In contrast, short MWNTs just showed the typical shear-thinning behaviour. Colloidal behaviour of diluted supra-NC suspensions. Photographs (left) of MWNT-COOH/DMF, supra-MWNT/DMF droplets on a SiO2surface after drying at 20 °C (b) and 100 °C (c). In (b), the supra-MWNTs in water-added suspension droplets move towards the edge because the QHB was destroyed by water molecules. The right schematic illustration shows the colloidal behaviour of MWNTs-COOH and supra-MWNTs during drying in the liquid droplets. (d) FESEM images of the As-prepared GO obtained using the homogenizer and small GO nanoplatelets broken by horn sonication (200 W, 20 kHz). Scale bar, 2 μm. (e) Schematic illustration of the unstable dispersion of the small RGO sheets through partial QHB networking. (f) Photographs of the reduced small GO suspension in DMF after the introduction of UHP motifs showing an unstable dispersion. Figure 2: Rheological and colloidal evidence of network formation. ( a ) Shear viscosity plot for supra-NC pastes (~10 wt%) in DMF as a function of shear rate showing shear-thickening behaviour at a low shear rate. In contrast, short MWNTs just showed the typical shear-thinning behaviour. Colloidal behaviour of diluted supra-NC suspensions. Photographs (left) of MWNT-COOH/DMF, supra-MWNT/DMF droplets on a SiO 2 surface after drying at 20 °C ( b ) and 100 °C ( c ). In ( b ), the supra-MWNTs in water-added suspension droplets move towards the edge because the QHB was destroyed by water molecules. The right schematic illustration shows the colloidal behaviour of MWNTs-COOH and supra-MWNTs during drying in the liquid droplets. ( d ) FESEM images of the As-prepared GO obtained using the homogenizer and small GO nanoplatelets broken by horn sonication (200 W, 20 kHz). Scale bar, 2 μm. ( e ) Schematic illustration of the unstable dispersion of the small RGO sheets through partial QHB networking. ( f ) Photographs of the reduced small GO suspension in DMF after the introduction of UHP motifs showing an unstable dispersion. Full size image To further demonstrate the QHB effect on the dispersion of supra-NCs, we added water and HCl in a DMF solution as hydrogen-bond-breaking agents. To visualize the formation and breakage of QHBs, we observed the drying behaviour of dilute supra-MWNT (500 mg l −1 ) droplets on a substrate after adding distilled water and 0.01 wt% HCl diluted with DMF. Importantly, we observed the typical coffee-ring stain by comparing with that of supra-MWNTs suspended in pure DMF by increasing the amount of water in the supra-MWNT suspension (500 mg l −1 ) ( Supplementary Fig. S5 ). This indicates that QHBs are destroyed by water molecules. From the 30 vol% water solution, we observed significant aggregation of supra-MWNTs in dilute suspensions because of the increased van der Waals interactions between the CNT side walls caused by the solubility parameter mismatch. However, we observed that large supra-MWNT aggregates were suspended without precipitation, which occurs because of the solvation of the broken QHB motifs with DMF and water molecules. This means that the broken QHB motifs (UHP moieties) also aid the dispersion of CNTs in DMF as well as the formation of networks by the QHB motifs. However, dispersions of the supra-MWNT and supra-SWNT pastes were stable even upon the addition of up to 10 vol% water. This result indicates that the small amount of water does not completely destroy the multiple hydrogen bonds; they also do not have a detrimental effect on the solubility parameter matching. Thus, a small amount of hydrochloric acid (0.01 wt% in DMF) was added to the supra-MWNT suspension, which caused the supra-MWNTs to severely aggregate without precipitation even upon the addition of 1 ml of HCl (0.01 wt% in DMF) to 10 ml of supra-MWNT suspension (500 mg l −1 ). However, after drying on the substrate, the supra-MWNTs aggregated in the centre because of the stronger van der Waals interactions among the supra-MWNTs in the presence of HCl than that in the presence of water. Moreover, the supra-MWNT paste was unstable after the addition of HCl and is not printable, even by bar coating ( Supplementary Fig. S5d ). Furthermore, we found clear evidence for the fact that QHB networks significantly help in overcoming the van der Waals attractions between NC materials. Before the introduction of the QHB motifs, we broke the large graphene oxide (GO) nanoplatelets by high-energy horn sonication ( Fig. 2d ). The limited number of carboxylic acid groups at the large GO edge can be expected to be distributed in the small GO, as illustrated in Fig. 2d because the horn sonication cannot further introduce carboxylic acid groups. Therefore, the small GO consisting of a smaller number of carboxylic acid groups cannot be interconnected with each other. Most importantly, we found that the small RGO did not form stable dispersions in the paste ( Fig. 2f ) because of the lack of interconnection through the QHB moieties, as illustrated in Fig. 2e , whereas the large supra-GO platelets reduced by hydrazine (supra-RGO) formed well-dispersed conducting paste by overcoming the van der Waals interactions between the RGO nanosheets, as illustrated in Fig. 1 . Therefore, we believe that the QHBs between the attached UHP moieties stabilize the concentrated colloidal dispersion of NC materials by overcoming the van der Waals interactions between the NC materials. Electrical and structural characteristics of printed supra-NCs Highly conductive NC electrodes are attractive both for printed electronics and for electrochemical applications. Therefore, we measured the electrical conductivities of the printed supra-NC and supra-NC hybrid films ( Fig. 3a ). The electrical conductivity of the supra-LMWNT film reaches 6,000 S m −1 . To further improve the electrical properties of the supra-LMWNT film, commercially available Ag NWs were used as highly conductive one-dimensional (1D) networking agents. Previously, 1D Ag NWs have been used to electrically modify two-dimensional (2D) graphene films [23] , [24] . In our study, the electrical conductivity of the supra-LMWNT film ( Fig. 3e ) dramatically improved from ~6,000 to ~500,000 S m −1 after hybridization with Ag NWs (5 vol%) ( Fig. 3f ). Moreover, the electrical conductivity of the supra-SWNT film ( Fig. 3g ) was dramatically enhanced from ~22,000 to ~100,000 S m −1 by the addition of a polymerized TiO 2 sol ( Fig. 3h ), which induced significant p-type doping as demonstrated the significant blue shift (~10 cm −1 ) of the G-band observed in the Raman spectrum ( Fig. 3b ) [25] . Notably, the supra-SWNT/RGO hybrid film ( Fig. 3k ) showed a high electrical conductivity of ~25,000 S m −1 , which is slightly higher than those of the supra-SWNT film (~22,000 S m −1 ) and the supra-RGO coating (~20,000 S m −1 ) ( Fig. 3j ). These electrical conductivities are larger than that (10,000 S m −1 ) reported in the literature for a printing process [3] . Disregarding the printing process, the electrical conductivity of the SWCNT/RGO hybrid film is slightly superior to that reported for graphene/conducting polymer composite films prepared by spin coating for transparent electrode applications [26] . The electrical conductivity of the TiO 2 -doped supra-SWNT film corresponds to that of the transparent SWNT film doped with F4TCNQ that was fabricated by spray coating with SWNT dispersion in NMP (110,000 S m −1 ) [27] . 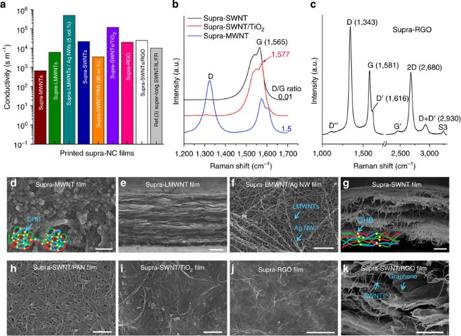Figure 3: Electrical and structural characteristics of supra-NCs. (a) Electrical conductivities of films fabricated via bar coating of a colloidal NC suspension stabilized by QHB networks along with previously reported values for a super-long SWNT/ionic liquid (IL)/fluorinated rubber (FR) hybrid film3for comparison. (b,c) Raman spectra of supra-MWNTs, supra-SWNT film and supra-SWNT/TiO2hybrid film (withλEX=633 nm) (b), and supra-RGO film (withλEX=532 nm) (c). FESEM micrographs of the surfaces or cross-sections of the printed films, prepared with (d) supra-MWNTs (scale bar, 5 μm), (e) long supra-MWNTs (scale bar, 10 μm), (f) long supra-MWNTs/Ag NWs (95/5 v/v) (scale bar, 1 μm), (g) supra-SWNTs (scale bar, 1 μm), (h) supra-SWNTs/polyacrylonitrile (PAN) (70/30 w/w) (scale bar, 500 nm), (i) supra-SWNT/TiO2sol (1/1 w/w) (scale bar, 500 nm), (j) supra-RGO (scale bar, 5 μm) and (k) supra-SWNT/RGO (1/1 w/w) (scale bar, 1 μm). MWNTs and SWNTs are interconnected by the QHB motifs, as schematically shown in (d) and (g), forming microballs and a layered structure, respectively. Figure 3: Electrical and structural characteristics of supra-NCs. ( a ) Electrical conductivities of films fabricated via bar coating of a colloidal NC suspension stabilized by QHB networks along with previously reported values for a super-long SWNT/ionic liquid (IL)/fluorinated rubber (FR) hybrid film [3] for comparison. ( b , c ) Raman spectra of supra-MWNTs, supra-SWNT film and supra-SWNT/TiO 2 hybrid film (with λ EX =633 nm) ( b ), and supra-RGO film (with λ EX =532 nm) ( c ). FESEM micrographs of the surfaces or cross-sections of the printed films, prepared with ( d ) supra-MWNTs (scale bar, 5 μm), ( e ) long supra-MWNTs (scale bar, 10 μm), ( f ) long supra-MWNTs/Ag NWs (95/5 v/v) (scale bar, 1 μm), ( g ) supra-SWNTs (scale bar, 1 μm), ( h ) supra-SWNTs/polyacrylonitrile (PAN) (70/30 w/w) (scale bar, 500 nm), ( i ) supra-SWNT/TiO 2 sol (1/1 w/w) (scale bar, 500 nm), ( j ) supra-RGO (scale bar, 5 μm) and ( k ) supra-SWNT/RGO (1/1 w/w) (scale bar, 1 μm). MWNTs and SWNTs are interconnected by the QHB motifs, as schematically shown in ( d ) and ( g ), forming microballs and a layered structure, respectively. Full size image Basically, the electrical conductivity of the CNT network films depends on the crystalline structure of the CNTs. The intensity ratio of the G and defect D bands ( I D / I G ) in the Raman spectrum is related to the sp 2 carbon cluster sizes in the CNTs and is nearly proportional to the defect density [28] . It is worth noting that D/G ratio of the SWNTs was dramatically decreased from 0.05 to 0.01, whereas that of the MWNTs was slightly decreased from 1.6 to 1.5 ( Fig. 3b ). This can be attributed to the removal of the amorphous carbonaceous materials and the opening of the end caps of the pristine SWNTs during the QHB formation process without defect formation on the nanotube surface. The small I D / I G value of the supra-SWNTs indicates that the QHB groups may be attached mostly at the ends of the highly crystalline SWNTs, not on the side walls. The increase in organic moieties after the coupling reaction was confirmed by the thermogravimetric analysis ( Supplementary Fig. S6 ). A greater percentage of QHB motifs (~8% increase) was attached to the MWNTs than to the SWNTs (~2 wt% increase) because the defective side walls of the MWNTs synthesized by chemical vapour deposition are more reactive than those of the SWNTs synthesized by arc discharging during acid treatment [29] , [30] . Moreover, it is apparent that a low density of QHB motifs attached to the ends of the SWNTs synergistically affects the dispersion of the SWNTs in DMF to overcome the van der Waals interactions between the SWNTs. In particular, supra-RGO nanoplatelets had a high-intensity ( I 2D / I G ~1.0), narrow (full width at half maximum ~55.9 cm −1 ) 2D band peak ( Fig. 3c ), suggesting that it has a more ideal graphitic structure than other RGO samples with a high defect concentration ( Supplementary Fig. S7 ) [31] . The small D'/G (0.417) and S3/2D (0.203) intensity ratios also demonstrate the formation of high-quality graphene nanoplatelets [32] . These results of the Raman studies confirm the origin of the high electrical conductivities of our conducting pastes. To correlate the structural characteristics of the supra-CNTs with the morphology of the supra-CNT microstructures, we observed the surface and cross-section of the supra-CNT samples using scanning electron microscopy. The supra-MWNTs showed interconnected assembled microball structures ( Fig. 3d ), which have not been observed previously in functionalized MWNT samples. In the case of the supra-LMWNTs and the supra-SWNTs, 2D-assembled CNT mats ( Supplementary Fig. S8 ) were observed, which were stacked into unusual layered structures in the coated film ( Fig. 3e,g ). This layered structure may contribute to the relatively strong shear-thickening behaviour of the supra-SWNT and the supra-LMWNT pastes, which was similar to that of the 2D supra-RGO nanoplatelets ( Fig. 2a ). This behaviour can be attributed to the π–π interactions between the unfunctionalized side walls. The morphological differences between the supra-MWNTs and supra-SWNTs result from the positioning of the QHB motifs (yellow dots), as schematically shown in Fig. 3e,f , because defective MWNT surfaces and the ends of the SWNTs are easily functionalized by mild acid treatments. Electrochemical applications of printed supra-NC films Potential energy-related applications of the printed supra-NC electrodes were demonstrated using homogeneously distributed supra-SWNT/RGO hybrid ( Fig. 3k ) and supra-MWNT pastes as alternative electrochemical electrodes in electrochemical capacitors and DSCs, respectively. First, the supra-SWNT/RGO hybrid electrode was used in electrochemical capacitors, which store energy through either ion adsorption (electrochemical double-layer capacitors) or fast surface redox reactions (pseudo-capacitors). The cyclic voltammetry (CV) curves acquired at increasing scan rates from 10 to 1,000 mV s −1 in 1 M H 2 SO 4 solution ( Fig. 4a ) indicated that the devices acted as nearly ideal electrochemical capacitors [33] , [34] , [35] . Analysis of the CV curves showed that the supra-SWNT/RGO hybrid electrode exhibits a high specific capacity ( C sp ) of 217 F g −1 at 10 mV s −1 , which was significantly retained at 90.3% even at the extremely high scan rate of 1,000 mV s −1 ( C sp =196 F g −1 ) ( Fig. 4b ). The impedance spectrum acquired, shown as a Nyquist plot in Fig. 4c , exhibited a typical arc in the high-frequency region and a spike in the low-frequency region. Notably, the Nyquist plot shows an almost vertical line at low frequencies, indicating highly capacitive behaviour. The superior rate capability and excellent capacitive behaviour of the supra-SWNT/RGO hybrid electrode can be attributed to the effective redox reaction on the supra-SWNT/RGO surface with QHB motifs and residual oxidative groups [36] and to the high electrical conductivity (~25,000 S m −1 ) of the supra-SWNT/RGO electrode. The excellent interfacial contact afforded by the π – π interactions between the SWNTs and the graphene nanoplatelets facilitates the fast transfer of electrons throughout the whole electrode matrix. 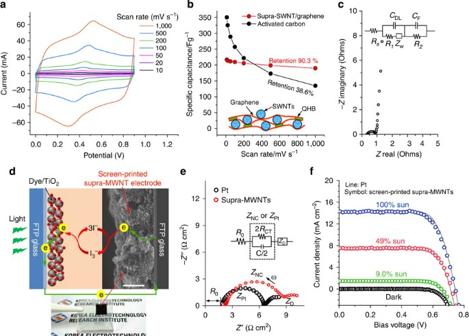Figure 4: Electrochemical performance of supra-NC materials. (a) Cyclic voltammograms of supra-SWNT/RGO hybrid electrodes printed on Ti taken at different scan rates in 1 M H2SO4electrolyte. (b) Specific capacitance (Csp) of supra-SWNT/RGO and commercial activated carbon electrodes for comparison as a function of increasing scan rate from 10 to 1,000 mV s−1. The inset in (b) shows a schematic illustration of a cross-sectional view of the supra-SWNT/RGO hybrid electrode. (c) Electrochemical impedance plot of the supra-SWNT/RGO hybrid electrode. The spectrum was taken in 1 M H2SO4in a frequency range from 100 kHz to 100 mHz. A Randles equivalent circuit representing the circuit elements for the Nyquist plot is shown in the inset.RSis the solution resistance,R1is the ionic charge-transfer resistance,R2is the electron-transfer resistance,CDLis the double-layer capacitance,CFis the bulk faradaic pseudocapacitance andZwis the diffusion-controlled Warburg impedance. (d) Schematic representation of a DSC, in which the screen-printed supra-MWNT pattern on FTO glass used as a cathode is shown as a real side-view SEM image. Scale bar, 5 μm. Photo image shows a real picture of a screen-printed supra-MWNT electrode. (e) RCT at the interface between the supra-MWNT-based cathode material and the electrolyte. (f) Comparison of J-V curves for Pt and supra-MWNTs counter electrodes in DSCs. Figure 4: Electrochemical performance of supra-NC materials. ( a ) Cyclic voltammograms of supra-SWNT/RGO hybrid electrodes printed on Ti taken at different scan rates in 1 M H 2 SO 4 electrolyte. ( b ) Specific capacitance ( C sp ) of supra-SWNT/RGO and commercial activated carbon electrodes for comparison as a function of increasing scan rate from 10 to 1,000 mV s −1 . The inset in ( b ) shows a schematic illustration of a cross-sectional view of the supra-SWNT/RGO hybrid electrode. ( c ) Electrochemical impedance plot of the supra-SWNT/RGO hybrid electrode. The spectrum was taken in 1 M H 2 SO 4 in a frequency range from 100 kHz to 100 mHz. A Randles equivalent circuit representing the circuit elements for the Nyquist plot is shown in the inset. R S is the solution resistance, R 1 is the ionic charge-transfer resistance, R 2 is the electron-transfer resistance, C DL is the double-layer capacitance, C F is the bulk faradaic pseudocapacitance and Z w is the diffusion-controlled Warburg impedance. ( d ) Schematic representation of a DSC, in which the screen-printed supra-MWNT pattern on FTO glass used as a cathode is shown as a real side-view SEM image. Scale bar, 5 μm. Photo image shows a real picture of a screen-printed supra-MWNT electrode. ( e ) RCT at the interface between the supra-MWNT-based cathode material and the electrolyte. ( f ) Comparison of J-V curves for Pt and supra-MWNTs counter electrodes in DSCs. Full size image For further examination of the performance of our supra-NC films, screen-printed supra-MWNT electrodes on a fluorine-doped tin oxide (FTO) substrate were applied as electrochemical electrodes in DSCs ( Fig. 4d ). The alternative supra-MWNT-based cathode provided photovoltaic performance improvements similar to those provided by conventional Pt nanoparticles ( Fig. 4f ; Supplementary Table S1 ). The charge-transfer resistance (RCT) at the interface between the supra-MWNT cathode material and the electrolyte could be roughly estimated from an equivalent electrical circuit ( Fig. 4e ) [37] . The supra-MWNT-based electrodes showed two characteristic peaks: one at a high frequency above 10 kHz ( Z network or Z pore ) [38] and one in the mid-frequency range near 10 Hz ( Z NC ). The latter was mainly related to the electrochemical performance of the electrodes. The RCT (3.15 cm 2 ) derived from the Z NC of the supra-MWNT surface was slightly higher than that (2.37 cm 2 ) derived from the impedance at the Pt electrode ( Z Pt ). Based on the previously suggested value of RCT=2–3 Ω cm 2 , this result indicates that the supra-MWNT electrode functioned as a good cathode and enabled the efficient reduction of I 3– to I − in the DSCs [39] . The supramolecular methods reported here represent concepts for realizing NC materials with much higher level of processability and chemical compatibility compared with conventional methods. In the case of multiple hydrogen bonds employed in this study, the macroscopic structure and rheological properties of the colloidal system can be manipulated by the supramolecular assembly of nanoparticles having a variety of dimensions. We demonstrated that a dispersant-free NC paste could be prepared by introducing QHB motifs into NC materials, such as MWNTs, SWNTs and graphene nanoplatelets. One of the advantages of our strategy is that it is easy to convert the multiple hydrogen-bonded supramolecular structure into commercially available NC materials even on a large scale. The properties of the resulting supra-NC materials can also be easily tuned by changing the ratio of NC materials and the amount of carboxylic acid groups by acid treatment. A high chemical compatibility of supra-NC pastes could contribute to the broad applications of NC-based pastes. The field in which supramolecular chemistry and NC material science meet can be developed into a vast area of research and technology development, ranging from the assembly of NC particles to flexible conducting film and fibre technologies. We hope our study will promote further practical work on the conducting pastes based on NC materials. Materials Pristine short/long MWNTs (produced by chemical vapour deposition, Hanwha Nanotech) and SWNTs (produced by arc discharging, Nanosolutions) were functionalized with carboxylic acid using a mixture of sulphuric acid and nitric acid (7:3 v/v) at low temperature, 50 °C to minimize the defect formation in the starting materials; the acid treatment conditions were optimized by varying the treatment time from 12 to 36 h ( Supplementary Figs S1 and S2 ). GO was synthesized using a modified Brodie method [34] . Pure graphite (Alfa Aesar, 99.999% purity, –200 mesh) was mixed with fuming nitric acid and sodium chlorate at room temperature with stirring for 48 h. After acid treatment, the product was purified by washing, filtering and cleaning. The synthesized graphite oxide powder was immersed in aqueous KOH at pH 10 to a concentration of 2 g l −1 , and exfoliation and dispersion were carried out by using homogenizer for 1 h to minimize the defect formation [35] . Subsequently, the aging process was performed to attach K + ions on the graphene basal plane by using rotary evaporator for 2 h, and excess K + ions were removed by centrifugal washing several times. The resulting mixture was centrifuged and freeze-dried to obtain the dispersible GO powder. The resulting GO powder was then dispersed in DMF by bath sonication for 30 min. ( Supplementary Fig. S9 ) The supra-GO paste was reduced by adding hydrazine monohydrate (N 2 H 4 ) to reach a final concentration of 4 mM, followed by heating at 100 °C for 10 h. Synthesis of the supra-NCs having quadruple hydrogen bond networks The supra-NCs were synthesized in three steps from NCs functionalized with carboxylic acid groups (NCs-COOH), TDI (Aldrich) and AHMP (Aldrich) as shown in Fig. 1a . The CNTs were functionalized with carboxylic acid using a mixture of sulphuric acid and nitric acid (7:3 v/v) at low temperature, 50 °C to minimize the defect formation in the starting materials. The less defective and single-layered GO nanoplatelets having carboxylic acid were synthesized using a modified Brodie method [40] , [41] . First, 2.0 g of NCs-COOH were dispersed in 800 ml DMF by bath sonication for 1 h under argon purging. The isocyanate groups were attached using the coupling reaction by adding an excess amount (4 ml) of TDI to the NC suspension, following by heating at 50 °C for 24 h. The unreacted TDI molecules were removed by washing and vacuum filtration. The 2 g of isocyanate-modified NCs thus obtained was then redispersed in 800 ml DMF by bath sonication. AHMP (1.8 g) and 4 ml triethylacetate (catalyst) were added to the solution to attach the UHP moieties, and the solution was heated at 100 °C for 20 h under magnetic stirring. The modified NC materials were then purified by centrifugation and vacuum filtration to remove the unreacted agents, and the product was characterized ( Supplementary Figs S3–S5 ). The supra-NC pastes were then prepared simply by mixing the supra-NC powder and organic solvents using a rotary mixer. The supra-GO paste was reduced by adding hydrazine monohydrate (N 2 H 4 ) to reach a final concentration of 4 mM, followed by heating at 100 °C for 10 h. Chemical compatibility of the supra-NC materials For hybridization of NC materials, polyacrylonitrile and AgNO 3 were purchased from Aldrich. Polymerized TiO 2 precursor sol was prepared using titanium isopropoxide/acetylacetone (in a 1:5 molar ratio), ethanol, HCl and water by stirring at 60 °C for 10 h, followed by solvent exchange with DMF [21] . We investigated the chemical compatibility of the supra-NCs, which is one of the most important characteristics of conducting pastes, by hybridizing the supra-NCs with a polymer, metal or metal oxide material in solution ( Supplementary Fig. S10 ). First, the mechanical and electrical properties of the SWNT coatings were improved by hybridizing a polymerized TiO 2 precursor sol (mixture of titanium isopropoxide and acetylacetone) in DMF and the supra-SWNTs. Second, supra-CNTs were hybridized with polyacrylonitrile to a concentration of over 70 wt% CNTs using a simple mixing process. Flexible conducting fibres were fabricated from the prepared paste by a solution-spinning process using a water/ethanol (1/1 v/v) mixture as a coagulation bath. Third, Ag was selectively attached to the surfaces of the supra-MWNTs in DMF solution using an AgNO 3 precursor that reacted with the amide bonds of the QHB motifs. Moreover, aqueous suspension of Ag NWs (diameter ~35 nm, length ~25 μm) purchased from Nanopyxis were directly mixed with a long supra-MWNT paste to enhance the electrical conductivity ( Supplementary Fig. S11 ). Before mixing, the water in the Ag NW suspension was evaporated and replaced with DMF to minimize the detrimental effects of water on the dispersion stability of super-CNT pastes. The presence of Ag in the supra-CNT/Ag NW and supra-CNT/Ag hybrid films was characterized by energy-dispersive spectroscopy and X-ray diffraction. Electrochemical characterization The supra-SWNT/RGO hybrid paste was thinly coated on a carbon-adhesive-supported Ti substrate and dried at 200 °C for 1 h. As a control sample, the high-grade commercially activated carbon powder (MSP20, Kansai Cokes Chem. ), polyvinylidene difluoride (MSP20 contrast 7%) in N -methyl-2-pyrrolidone were mixed and deposited on the Ti substrate. For the three electrode system, a Pt plate and a saturated calomel electrode were used as counter and reference electrodes, respectively. The electrolyte used was 1 M H 2 SO 4 . The electrochemical performance of the electrode was measured using a potentiostat (Bio-Logic SAS, VSP/Z-01, France). The CV test of the cell was performed from 0 to 0.9 V. Electrochemical impedance spectroscopy measurements were carried out over a frequency range of 100–0.1 kHz. All electrochemical tests were performed at room temperature. The specific capacitance of the film electrode was calculated from the voltammetric charge using the CV curve in Fig. 4a according to equation (1): where C p, i , m and ΔE are the specific capacitance of the film electrode, the instantaneous current in cyclic voltammograms, the mass of the deposited supra-SWNT/RGO hybrid film and the potential window ( ΔE=E 2 −E 1 ), respectively. Fabrication and characterization of DSCs A TiO 2 photoanode was fabricated to have a double-layer structure composed of a transparent nanoporous layer 14 μm thick and a scattering layer 6 μm thick, deposited on FTO glass (TEC8, sheet resistance 8–9 ohm/square, Pilkington). This structure is conventionally used in conjunction with the N719 dye, (Ru(II)LL′(NCS) 2 (L=2,2′-bipyridyl-4,4′-dicarboxylate, L′=2,2′-bipyridyl-4,4′-dicarboxylate ditetrabutylammonium), Solaronix). TiO 2 pastes were purchased from JGC Catalysts and Chemicals and screen-printed on the FTO glasses. The printed TiO 2 layers were annealed at 480 °C for 1 h and immersed in a 0.3-mM N719 ethanol solution for 21 h at room temperature. The supra-MWNT paste was applied on FTO glass by screen printing and the printed layers were treated at 250 °C for 1 h in air. The printed supra-MWNT pattern was formed via screen printing with a patterned screen mask (SUS 200 mesh) on FTO glass plates fixed on the vacuum chuck. The patterned screen mask was prepared by using a photoresist that is highly resistant to chemicals: DMF was used to disperse the supra-NCs in this study. Moreover, before printing, the FTO glass was treated with UV–ozone for 2 min to improve adhesion between the supra-MWNT paste and the FTO substrate. For reference cells, Pt catalytic layers were thermally prepared on FTO substrates with Pt paste (Solaronix) at 400 °C for 30 min. The stained TiO 2 photoanode and the prepared MWNT or thermally platinized counter electrodes were assembled with a 60-μm-thick hot-melt film (Surlyn, Solaronix) to produce a sandwich-type cell. The liquid electrolyte consisted of 0.8 M 1-butyl-3-methylimidazolium iodide (BMImI, TCI), 0.2 M 1,3-dimethylimidazolium iodide (C-TRI), 0.05 M LiI (Aldrich), 0.07 M iodine (Aldrich), 0.1 M guanidine thiocyanate (Aldrich) and 0.5 M 4- tert -butylpyridine (Aldrich) in acetonitrile. The cell was filled with the liquid electrolyte through a hole by vacuum backfilling, and the hole was sealed with a cover glass. Photocurrent−voltage ( J − V ) characteristics were obtained using a Keithley model 2,400 source measure unit. The irradiation source was a 300 W Xenon lamp on an Oriel solar simulator with an air mass 1.5-G filter. The power of the solar simulator was calibrated using an NREL-calibrated Si solar cell equipped with an IR-cutoff KG-5 filter. The illuminated area of the cell was defined by a black mask with an aperture area of 0.2025, cm 2 , smaller than the diameter of the stained TiO 2 , in order to eliminate diffuse light from the transparent glass substrate. Electrochemical characterizations were performed using a Princeton Applied Research Potentiostat 2273. Impedance spectra were measured using symmetrical sandwich dummy cells fabricated in the same manner as the DSCs, except for the presence of two identical electrochemical electrodes. The spectra were acquired at a bias voltage of 100 mV to avoid the mass transfer-controlled region. The modulation amplitude was 10 mV over the frequency range from 100 kHz to 100 mHz. EIS data were processed using the ZSimpWin software. Characterization of the supra-NC materials The surfaces and cross-sectional morphologies of the samples were imaged using field-emission scanning electron microscopy (HITACHI S4800). The structural characteristics of the pristine CNT powder and supra-NCs and supra-SWNT/TiO 2 hybrid films were investigated using confocal Raman spectrometry (NTEGRA SPECTRA, NT-MDT) with excitation wavelengths of 532 and 633 nm, respectively. The functional groups of the NCs-COOH and supra-NCs were assigned by XPS, and FTIR spectroscopy using a Multilab2000 (Thermo VG Scientific Inc.) spectrometer with monochromatized Al K X-ray radiation as the X-ray excitation source and an FTIR spectrometer (JASCO, Model 4200UP), respectively. The quantities of organic moieties in each synthesis step were confirmed by the thermogravimetric analysis (TA Instruments, TGA Q500). The shear viscosities of the supra-NC pastes were measured using a Brookfield viscometer (DV-111 ultra). The electrical conductivity was measured by the four-point probe method (Keithley, 2000 Multimeter) at room temperature. How to cite this article: Han, J. T. et al . Dispersant-free conducting pastes for flexible and printed nanocarbon electrodes. Nat. Commun. 4:2491 doi: 10.1038/ncomms3491 (2013).